IgGs are made for walking on bacterial and viral surfaces Binding of antibodies to their cognate antigens is fundamental for adaptive immunity. Molecular engineering of antibodies for therapeutic and diagnostic purposes emerges to be one of the major technologies in combating many human diseases. Despite its importance, a detailed description of the nanomechanical process of antibody–antigen binding and dissociation on the molecular level is lacking. Here we utilize high-speed atomic force microscopy to examine the dynamics of antibody recognition and uncover a principle; antibodies do not remain stationary on surfaces of regularly spaced epitopes; they rather exhibit ‘bipedal’ stochastic walking. As monovalent Fab fragments do not move, steric strain is identified as the origin of short-lived bivalent binding. Walking antibodies gather in transient clusters that might serve as docking sites for the complement system and/or phagocytes. Our findings could inspire the rational design of antibodies and multivalent receptors to exploit/inhibit steric strain-induced dynamic effects. The high specificity of antibodies for their cognate antigens is a paradigm for molecular recognition. Besides its biological function as part of the adaptive immune system, antibody–antigen recognition is exploited for labelling and purification in biochemistry, molecular biology and bio-inspired nanotechnology [1] . Engineered antibodies are used for therapeutic [2] and diagnostic purposes [3] for treating cancer and autoimmune and infectious diseases. In immunoglobulin G (IgG), an Fc stem connects two identical Fab arms resulting in a Y-shaped molecule with C2-symmetry. IgGs are considered molecular calipers [4] as they can attach adjacent epitopes [5] within a distance of roughly 6–12 nm (refs 6 , 7 ). The Fc stem is recognized by the complement system [8] and by phagocytic cells [9] . The antigen encounter process typically starts with the binding of one Fab to an epitope on the surface on an antigen. The second Fab explores the surrounding space until it establishes an additional connection to the antigen by binding to another epitope [10] . To a first approximation, bidentate binding to two symmetry-related epitopes, as are present on the surface of many pathogens, should be stabilized by twice the activation energy barrier (Δ G 0 ) of a monovalent bond. This is indeed found when surface antigens are either embedded in a fluid lipid membrane or are part of a flexible matrix and thus possess high lateral mobility facilitating stress-free bivalent binding of IgG molecules. However, naked viruses and a great number of prokaryotes, including numerous human and animal pathogens [11] , possess a quasi-crystalline surface coat with the antigens arranged on a rigid lattice. Therefore, bivalent binding of IgG is likely to inflict steric strain [12] . Here, we studied binding of monoclonal IgG1 antibodies (MAb) to various two-dimensional (2D) crystalline protein layers and to a viral capsid using high-speed atomic force microscopy (HS-AFM) [13] that acquires images within tens of milliseconds (as compared with minutes with conventional AFM), allowing for real time recording of molecular processes [14] , [15] , [16] , [17] , [18] , [19] . HS-AFM imaging of IgG bound to bacterial and viral surfaces revealed that (i) the antibodies were rapidly walking around on a time scale of 0.01–1 s/step, (ii) this time varied with the distance and the orientation of the antigenic sites with respect to each other, (iii) except from rarely occurring complete dissociation, the antibodies remained bound with at least one Fab arm and (iv) even at moderate antibody density transient clusters were formed. Stochastic walking of IgGs on patterned antigenic epitopes We first studied the behaviour of antibodies on a modified purple membrane from Halobacter salinarium where, similar to bacterial surfaces, the cognate epitopes are laterally and orientationally confined. HS-AFM imaging ( Fig. 1a ) of the cytoplasmic face of these membranes revealed the characteristic trigonal lattice structure of bacteriorhodopsin trimers (unit cell: a = b =6.2 nm; γ =120°) carrying the carboxyl-terminal amino acid sequence of the L protein antigen of Sendai virus (Sendai PM). Each bacteriorhodopsin monomer displays one epitope (in its cytoplasmic EF loop) representing a high-affinity target for the monoclonal mouse IgG 1 MAb VII-E-7 (refs 20 , 21 ). Antibodies bound to Sendai PM ( Supplementary Movie 1 , 1.25 frames s −1 per second) did not remain stationary but moved around on the surface ( Supplementary Movie 2 ). Black arrows in Fig. 1c point to the approximate positions of the two Fab arms of an individual IgG molecule as a function of time, taking into account the IgG geometry and the conformations observed. Note that the Fc part is invisible because of its highly flexible connection with the Abs hinge region. In consecutive images, only one out of the two Fab arms was seen to change its position (indicated with red arrows), while the other one remained fixed (white arrows). This erratic ‘bipedal locomotion’ is generated by detachment of one Fab arm followed by reattachment to an adjacent epitope. In some instances, the antibody remained in the identical conformation for up to one second (two white arrows between successive images). The cartoon ( Fig. 1b ) illustrates this motion and the corresponding centre-of-mass (COM) trajectory (black arrows) of the antibody. For quantification, trajectories of molecules were generated by connecting COMs in the image series ( Supplementary Movie 3 , inset Fig. 2a ) and the set of trajectories was then analysed with respect to step size ( Fig. 2a ). Dwell times were derived from the number of consecutive images in which individual antibodies remained stationary ( Fig. 2b ). The cumulative distribution ( Fig. 2b inset) follows a monoexponential curve with a time constant of 0.519±0.022 s. The trajectories were further subjected to a mean square displacement analysis (MSD, cf . Methods) that revealed a linear dependence. This behaviour is well known to reflect a non-directional, random-like movement. The apparent diffusion constant of this movement on Sendai PM was D =6.1±0.4 nm 2 s −1 ( Fig. 2f , upper panel). As the MSD was linear and the AFM tip velocity did not impact on the time constant ( Supplementary Fig. 1 ), we conclude that the interaction between AFM tip and sample does not alter the antibody–antigen binding dynamics. 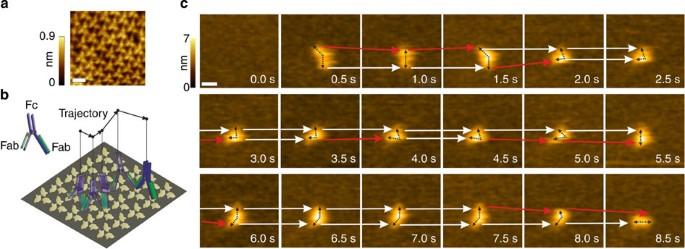Figure 1: Antibody locomotion on Sendai purple membrane. (a) Averaged AFM image (n=5) of the cytoplasmic face of Sendai PM. Scale bar, 10 nm. (b) Schematic of antibody locomotion. (c) Time series of AFM images showing an antibody moving on Sendai PM (Supplementary Movie 2). Att=0.5 s, an antibody appeared on the surface (projection of the Fab arms onto the PM surface is indicated by black arrows). The subsequent images show the same antibody with one or the other Fab arm in a different position (red arrow), while at least one Fab arm remains stationary between consecutive images (white arrows). Scale bar, 10 nm. Figure 1: Antibody locomotion on Sendai purple membrane. ( a ) Averaged AFM image ( n =5) of the cytoplasmic face of Sendai PM. Scale bar, 10 nm. ( b ) Schematic of antibody locomotion. ( c ) Time series of AFM images showing an antibody moving on Sendai PM ( Supplementary Movie 2 ). At t =0.5 s, an antibody appeared on the surface (projection of the Fab arms onto the PM surface is indicated by black arrows). The subsequent images show the same antibody with one or the other Fab arm in a different position (red arrow), while at least one Fab arm remains stationary between consecutive images (white arrows). Scale bar, 10 nm. 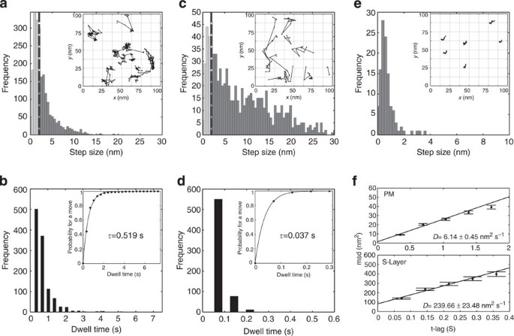Figure 2: Statistical analysis of antibody dynamics. (a) Distribution of step sizes in the trajectories (n=629) of individual anti-Sendai antibodies recorded on Sendai PM. Frame rate 3 frames s−1(Supplementary Movie 3). Dashed vertical line: threshold used for determining the dwell times. Inset: trajectories from that dataset. (b) Distribution of antibody dwell times. Inset: monoexponential fit to the cumulative distribution (τ=0.519 s). (c) Distribution of step sizes in the trajectories (n=102) of anti-Strep-Tag II antibodies recorded on S-layer. Frame rate 14 frames s−1(Supplementary Movie 4). Inset: trajectories from that dataset. (d) Distribution of antibody dwell times. Inset: monoexponential fit to the cumulative distribution (τ=0.037). (e) Distribution of step sizes in the trajectories (n=6) of anti-streptavidin antibodies recorded on a 2D streptavidin crystal. Frame rate 1.4 frames s−1(Supplementary Movie 6). Inset: trajectories from that dataset. (f) MSD versus t-lag of antibodies on PM (upper panel) and S-layer (lower panel). Antibodies perform a non-directional random-like walk on the regular epitope lattices with apparent diffusion constants (as determined from the slope of msd versus t-lag) of 6.1±0.4 nm2s−1and 239.7±23.5 nm2s−1, respectively (mean±s.d.). Full size image Figure 2: Statistical analysis of antibody dynamics. ( a ) Distribution of step sizes in the trajectories ( n =629) of individual anti-Sendai antibodies recorded on Sendai PM. Frame rate 3 frames s −1 ( Supplementary Movie 3 ). Dashed vertical line: threshold used for determining the dwell times. Inset: trajectories from that dataset. ( b ) Distribution of antibody dwell times. Inset: monoexponential fit to the cumulative distribution ( τ =0.519 s). ( c ) Distribution of step sizes in the trajectories ( n =102) of anti-Strep-Tag II antibodies recorded on S-layer. Frame rate 14 frames s −1 ( Supplementary Movie 4 ). Inset: trajectories from that dataset. ( d ) Distribution of antibody dwell times. Inset: monoexponential fit to the cumulative distribution ( τ =0.037). ( e ) Distribution of step sizes in the trajectories ( n =6) of anti-streptavidin antibodies recorded on a 2D streptavidin crystal. Frame rate 1.4 frames s −1 ( Supplementary Movie 6 ). Inset: trajectories from that dataset. ( f ) MSD versus t-lag of antibodies on PM (upper panel) and S-layer (lower panel). Antibodies perform a non-directional random-like walk on the regular epitope lattices with apparent diffusion constants (as determined from the slope of msd versus t-lag) of 6.1±0.4 nm 2 s −1 and 239.7±23.5 nm 2 s −1 , respectively (mean±s.d.). Full size image Antibody movement on a bacterial surface layer We then investigated the antibody movements on an S-layer protein of Lysinibacillus sphaericus CCM 2177 carrying the carboxyl-terminally fused peptide Strep-Tag II [22] , [23] . High-resolution topographs of the recombinant bacterial S-layer rSbpA-Strep-Tag II revealed identical non-glycosylated protein subunits (120 kDa), reassembled with a square (p4) lattice symmetry (lattice constant of a = b =13.1 nm; γ =90°; Supplementary Fig. 2a ). The Strep-tag II epitope, a high-affinity target for monoclonal anti-Strep-Tag II antibodies (StrepMAb-Immo) [24] , is located at the most prominent (flower like) protrusion [22] of the unit cell. Trajectories ( Fig. 2c , inset and Supplementary Fig. 2b ; Supplementary Movie 4 ) of anti-Strep-Tag II antibodies were collected and step size distribution ( Fig. 2c ) and the dwell times ( Fig. 2d ) were determined as above. The time constant (0.037±0.001 s; Fig. 2d , Supplementary Fig. 1 ) was more than one order of magnitude smaller than that for Sendai PM. MSD analysis of the trajectories yielded a non-directional, random-like movement with an apparent diffusion constant of D =239.7±23.5 nm 2 s −1 ( Fig. 2f , lower panel). Steric strain versus low affinity Dissociation of individual Fab arms of the antibody from their cognate epitopes might be caused either by low affinity or by steric strain impacting on the stability of the bond. The latter might originate from a mismatch in the geometry and/or symmetry of the epitope/paratope interactions that cannot be compensated for by the antibodies hinge region (that is, for example, non-ideal distance between the epitopes). Such effects are necessarily absent in monodentate binding. Therefore, we repeated the experiment in Fig. 2c ( Supplementary Movie 4 ) but used isolated anti-Strep-Tag II Fab fragments ( cf . Methods) instead of entire IgGs ( Supplementary Fig. 3 , Supplementary Movie 5 ). The monovalent Fab fragments appeared as round structures, remained stationary and did not dissociate within the time scale of the experiment (6 min). As Fabs are monovalent, this result proves that steric strain results from bivalent binding (and not from lack of affinity) and is the main driving force behind the observed antibody movement. The effect of epitope–paratope symmetry As demonstrated above, steric strain causes antibodies that bind via both Fab arms to move. Is there an arrangement of epitopes that allows for ‘relaxed’ (without steric strain) bivalent binding? In their equilibrium conformation [25] , antibodies exhibit twofold symmetry and can access epitope pairs within roughly 6–12 nm (refs 6 , 7 ). Streptavidin forms a rigid 2D crystal with twofold symmetry and a unit cell a = b =5.9 nm; γ =90° (refs 26 , 27 , 28 ); on supported lipid bilayers ( Supplementary Fig. 4a ); it provides ~19 epitope pairs along different crystal axes ( Fig. 3k ) that are within a suitable distance to allow for bivalent antibody binding. Nevertheless, almost all MAb bound to the streptavidin crystal in the same orientation along one of the crystal axes ( Supplementary Figs 4b and 5 ). This implies that they attached bivalently to epitope pairs with identical distance and symmetry ( Fig. 3k ) with the intrinsic Fab orientation being close to its equilibrium conformation ( Fig. 3b ). No movement was detected on the timescale of the experiment, indicating the absence of steric strain in this particular conformation of the bivalent antibody–antigen complex. Consequently, the trajectories of these static, bivalently bound antibodies ( Fig. 2e , inset) are strongly confined and originate from thermal drift only ( Supplementary Movie 6 ). The histogram of the step size of these trajectories ( Fig. 2e ) yielded a Gaussian-like distribution with about 2 nm in width reflecting solely the fluctuation of the Fc stem. Therefore, this value was used to set the threshold in the depiction of the steps analysed in Fig. 2a–d . Only when the epitope itself changed its position in the lattice, the antibody was forced to transiently bind to an epitope pair with other (presumably non-ideal) distance and (intrinsic) symmetry ( Supplementary Fig. 5 ). 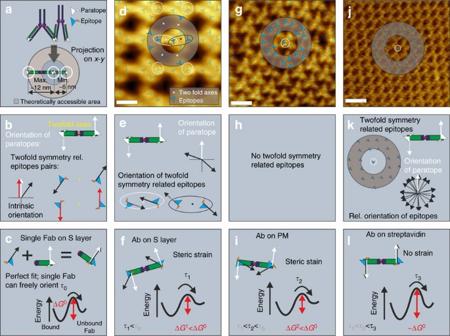Figure 3: Suboptimal spacing and orientation of epitope pairs makes IgG walk stochastically on antigenic surfaces. (a) On the binding of one of the two IgG Fab arms to an antigenic epitope the remaining arm can attach adjacent epitopes within a distance of roughly 6–12 nm6,7. (b) The paratopes exhibit twofold symmetry viewed down the IgG’s Fc axes (yellow asterisk). The paratopes intrinsic orientation with respect to the Fab arm represents an additional degree of freedom (projection on thex–yaxes; white arrows). Stress-free bivalent binding can be accomplished by binding to an epitope pair schematized by red arrows (orientations of white and red arrows match). In contrast, the epitope pair schematized as black arrows requires adjustment via rotation which might result in tension. (c) Single paratopes, as in the Fabs on the S-layer (Supplementary Fig. 3) can always fully adjust to a given epitope orientation. (d) Accessible epitope pairs on S-layer. Scale bar, 10 nm. (e) Twofold symmetry-related epitopes on S-layer. As we did not observe static bivalent binding, the intrinsic epitope orientations presumably did not match the intrinsic paratope orientation. (f) Dwell time (Fig. 2) of antibody residence on S-layers showed that the single bond lifetime (τ1) of a bivalently bound antibody is reduced when compared with the corresponding monovalently bound Fab. (g) Accessible epitope pairs on PM. (h) PM does not possess any twofold symmetry-related epitopes. Scale bar, 10 nm. (i) Steric strain in bivalent bound anti-Sendai antibodies lowers the energy barrier against thermal activation. (j) Accessible epitope pairs on a streptavidin crystal. Scale bar, 10 nm. (k) 22 2-fold related epitope pairs can be found within the accessible area, only differing in distance and intrinsic epitope orientation (cf. Methods). (l) At least one of these pairs allows for bivalent binding with negligible strain resulting in static bivalent binding (cf.Fig. 2e). Figure 3: Suboptimal spacing and orientation of epitope pairs makes IgG walk stochastically on antigenic surfaces. ( a ) On the binding of one of the two IgG Fab arms to an antigenic epitope the remaining arm can attach adjacent epitopes within a distance of roughly 6–12 nm [6] , [7] . ( b ) The paratopes exhibit twofold symmetry viewed down the IgG’s Fc axes (yellow asterisk). The paratopes intrinsic orientation with respect to the Fab arm represents an additional degree of freedom (projection on the x – y axes; white arrows). Stress-free bivalent binding can be accomplished by binding to an epitope pair schematized by red arrows (orientations of white and red arrows match). In contrast, the epitope pair schematized as black arrows requires adjustment via rotation which might result in tension. ( c ) Single paratopes, as in the Fabs on the S-layer ( Supplementary Fig. 3 ) can always fully adjust to a given epitope orientation. ( d ) Accessible epitope pairs on S-layer. Scale bar, 10 nm. ( e ) Twofold symmetry-related epitopes on S-layer. As we did not observe static bivalent binding, the intrinsic epitope orientations presumably did not match the intrinsic paratope orientation. ( f ) Dwell time ( Fig. 2 ) of antibody residence on S-layers showed that the single bond lifetime ( τ 1 ) of a bivalently bound antibody is reduced when compared with the corresponding monovalently bound Fab. ( g ) Accessible epitope pairs on PM. ( h ) PM does not possess any twofold symmetry-related epitopes. Scale bar, 10 nm. ( i ) Steric strain in bivalent bound anti-Sendai antibodies lowers the energy barrier against thermal activation. ( j ) Accessible epitope pairs on a streptavidin crystal. Scale bar, 10 nm. ( k ) 22 2-fold related epitope pairs can be found within the accessible area, only differing in distance and intrinsic epitope orientation ( cf . Methods). ( l ) At least one of these pairs allows for bivalent binding with negligible strain resulting in static bivalent binding ( cf . Fig. 2e ). Full size image The mechanism underlying antibody movement On binding of one of the two IgG Fab arms to an antigenic epitope, the remaining arm samples a ‘crown’ area of ~6 nm< r <~12 nm for symmetry-related epitopes [7] ( Fig. 3a ). Here, the paratopes exhibit a twofold symmetry when viewed down the IgG’s Fc twofold axis (yellow asterisk, Fig. 3b ). Because of the paratopes’ 3-D structure their orientation with respect to the Fab arm represents an additional degree of freedom (for simplicity we only consider its projection onto the x – y axis; white arrows, Fig. 3b ). Taking this into account, stress-free bivalent binding of an IgG within the accessible area requires (I) twofold symmetry of epitope pairs and (II) same intrinsic orientation of epitope pairs (with respect to the paratopes in the IgG). Both of these conditions are fulfilled by the epitope pair schematized by red arrows, Fig. 3b . The epitope pair schematized as black arrows exhibit twofold symmetry only; bivalent binding requires adjustment via rotation of the Fab around its axis, which might result in tension. A single antibody paratope, as represented by the Fabs on the S-layer ( Supplementary Fig. 3 ) can always fully adjust to a given epitope orientation. For dissociation of that single bond, the activation energy barrier, Δ G 0 , may be overcome by thermal energy within the bond lifetime τ 0 ( Fig. 3c ). The residence dwell time ( Fig. 2 ) of antibody on S-layers ( Fig. 3d ), showed that the single bond lifetime ( τ 1 ) of a bivalently bound antibody is reduced when compared with the corresponding monodentate Fab ( Supplementary Fig. 3 ). Since dissociation is governed by thermal energy, the reduction of bond lifetime is a consequence of a reduction of the underlying dissociation energy barriers (Δ G 1 , <Δ G 0 , Fig. 3f ). This latter is caused by steric strain resulting from the conformational adjustments necessary for bivalent attachment to epitope pairs that fail to comply with the geometric requirements described above ( Fig. 3a,b ). The ensuing accelerated dissociation of one Fab arm and its immediate rebinding to an adjacent site generates the stochastic movement observed in this study; while one Fab explores the environment similarly as reported for the initial antibody–antigen encounter process [10] , the other one remains attached. The role of the antibodies hinge region herein is twofold: on the one hand, it provides enough flexibility for the unbound Fab to probe for an epitope within a suitable distance, on the other hand it partly compensates steric strain in the bivalent bound state. Note that even though the S-layer comprises several twofold axes, only two pairs of twofold symmetry-related epitopes are within the area simultaneously accessible by both Fab arms. As we did not observe static bivalent binding, the intrinsic epitope orientations presumably did not match the intrinsic paratope orientation ( Fig. 3e ). On Sendai PM, twofold symmetry-related epitopes are not present at all ( Fig. 3g,h ). Thus, steric strain always occurs on bivalent antibody binding ( Fig. 3i ) resulting in antibody motions shown in Fig. 1c . Static bivalent antibody binding occurs more likely on antigenic surfaces exhibiting twofold symmetry and smaller distances between epitopes, like on a streptavidin crystal, providing a larger number (22) of twofold related epitope pairs within the accessible area ( Fig. 3j,l ). Each of these pairs only differs in distance and intrinsic epitope orientation with the latter almost equally distributed on the x – y plane ( Fig. 3k ). Thus, the probability for one of these epitope pairs allowing bivalent binding with negligible strain is higher, as it was indeed observed for anti-streptavidin antibodies on a streptavidin crystal. In this latter case, each of the bonds is stabilized through a dissociation energy barrier close to that of a monovalent bond, resulting in static bivalent binding ( Fig. 3l ). Antibodies form transient clusters As assessed through MSD analysis ( Fig. 2f ), antibodies are quite mobile on PM and S-layer as long as their surface density is low. However, at intermediate and high antibody densities, competition for the limited number of available epitopes alters their mobility resulting in an ensemble effect; despite of the individual antibodies moving quickly, aggregates are formed ( Fig. 4a ) in which motional freedom is significantly reduced ( Supplementary Movie 7 ). Due to a defect in the S-layer near the centre of the imaged region, a transient accumulation was repeatedly formed. This is seen in the time averages of the first and the second 100 frames (left and right panel in Fig. 4b ). Antibody aggregates of this size are required for binding of complement C 1q , a hexamer with a diameter of ~30–40 nm (ref. 29 ) ( Fig. 4c ). In fact, binding of C 1q to the S-layer surface of Gram negative bacteria and subsequent attachment of C 3b is known to ultimately result in clearance of the pathogens by phagocytes [9] . The high mobility of the antibodies within the plane of the bacterial surface may result in continuous growth of the docking region. This might facilitate Fc receptor-mediated phagocyte attachment. Similarly, phagocytes remove virions and immune complexes from the circulation [12] . 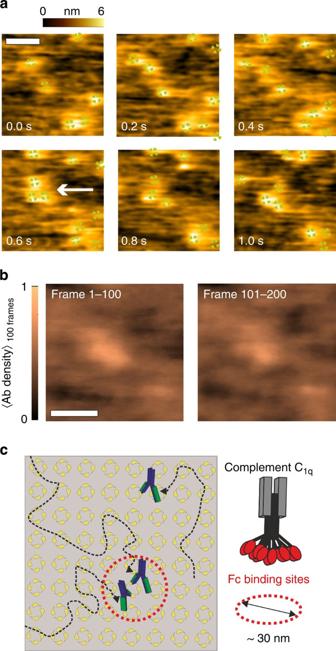Figure 4: Antibodies aggregate at moderate density. (a) Time series of AFM images of antibodies on S-layer (Supplementary Movie 7). Green marks indicate positions of individual antibodies. A transient accumulation appeared around the centre of the area at 0.6 s (arrow). Scale bar, 50 nm. (b) Averaged AFM images (n=100) taken fromt=0–20 s (left panel) andt=20–40 s (right panel) ofSupplementary Movie 7. The prominent density in the centre of both panels is the result of temporal clustering of several antibodies in 70–80% of the total measuring time. Scale bar, 50 nm. (c) As reported29, complement C1qbinds the Fc moiety of a single IgG only weakly. However, on accumulation of several Fc domains within a region of~30 nm (the diameter of C1q;red circle) the affinity of the hexameric C1qfor IgGs increases about a thousand fold. Figure 4: Antibodies aggregate at moderate density. ( a ) Time series of AFM images of antibodies on S-layer ( Supplementary Movie 7 ). Green marks indicate positions of individual antibodies. A transient accumulation appeared around the centre of the area at 0.6 s (arrow). Scale bar, 50 nm. ( b ) Averaged AFM images ( n =100) taken from t =0–20 s (left panel) and t =20–40 s (right panel) of Supplementary Movie 7 . The prominent density in the centre of both panels is the result of temporal clustering of several antibodies in 70–80% of the total measuring time. Scale bar, 50 nm. ( c ) As reported [29] , complement C 1q binds the Fc moiety of a single IgG only weakly. However, on accumulation of several Fc domains within a region of~30 nm (the diameter of C 1q; red circle) the affinity of the hexameric C 1q for IgGs increases about a thousand fold. Full size image Antibody dynamics on viral capsids Non-enveloped viruses exhibit patterned antigenic surfaces similar to those studied above except that the epitopes are arranged on a small and curved surface instead of a flat one. We studied the dynamics of two MAbs with different binding characteristics [30] on the surface of the common cold virus HRV-A2. Bivalent binding of monoclonal antibody 8F5 (ref. 6) [6] to symmetry-related epitopes on the viral capsid ( Fig. 5a ) followed dynamics ( Fig. 5b,d , Supplementary Movie 8 ) similar to that of antibodies on bacterial surfaces. Since the distance between adjacent epitopes is about 6 nm, a COM movement of roughly 3 nm was observed. In contrast, the movement of MAb 3B10 (ref. 31) [31] that only binds with one Fab arm is reminiscent of the wagging motion of single Fabs ( Fig. 5c,d ; Supplementary Movie 9 ). The absence of bivalent binding is due to the larger distance of the antigenic sites and/or to geometric constraints of the epitope/paratope interaction. In fact, 3B10 neutralizes HRV2 by crosslinking individual virions resulting in aggregation [32] . 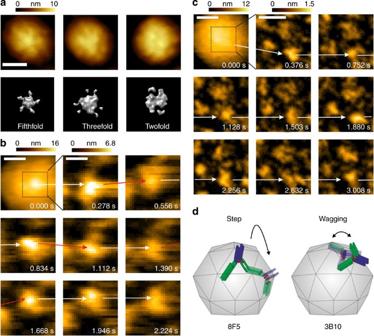Figure 5: Antibodies on human Rhino viruses. (a) Upper row: Averaged AFM images (n=5) of HRV2 particles with five, three and twofold symmetry axes of the icosahedral viral capsid (diameter=30 nm) facing upwards. Lower row: X-ray (PDB:1FPN) envelope of a virion viewed down each of the three symmetry axes. For better comparison with AFM images, only the upper 19 Å are depicted. Scale bar 10 nm. (b) Time series of AFM images (Supplementary Movie 8) of 8F5 IgG recorded on the surface of a single virion. Red arrows indicate a step, white arrows dwelling of the antibody between consecutive images. Scan size 25 × 25 nm2; scale bar, 10 nm. (first image), 12.5 × 12.5 nm2; scale bar 5 nm. (consecutive images; virus curvature in the original image was flattened: Colour scale range: 0–16 nm/0–6.8 nm. (c) Time series of AFM images (movie S9) of 3B10 IgG bound monovalently to the surface of a single virus. White arrows indicate dwelling of the antibody between consecutive images. Scan size and flattening as inb. (d) Schematics of the observed step-like motion of 8F5 (left) and wagging of 3B10 (right) on HRV2 (not to scale). Figure 5: Antibodies on human Rhino viruses. ( a ) Upper row: Averaged AFM images ( n =5) of HRV2 particles with five, three and twofold symmetry axes of the icosahedral viral capsid (diameter=30 nm) facing upwards. Lower row: X-ray (PDB:1FPN) envelope of a virion viewed down each of the three symmetry axes. For better comparison with AFM images, only the upper 19 Å are depicted. Scale bar 10 nm. ( b ) Time series of AFM images ( Supplementary Movie 8 ) of 8F5 IgG recorded on the surface of a single virion. Red arrows indicate a step, white arrows dwelling of the antibody between consecutive images. Scan size 25 × 25 nm 2 ; scale bar, 10 nm. (first image), 12.5 × 12.5 nm 2 ; scale bar 5 nm. (consecutive images; virus curvature in the original image was flattened: Colour scale range: 0–16 nm/0–6.8 nm. ( c ) Time series of AFM images (movie S9) of 3B10 IgG bound monovalently to the surface of a single virus. White arrows indicate dwelling of the antibody between consecutive images. Scan size and flattening as in b . ( d ) Schematics of the observed step-like motion of 8F5 (left) and wagging of 3B10 (right) on HRV2 (not to scale). Full size image Highly symmetric and repetitive antigenic epitopes are common to viruses and bacteria and are almost universal in Archaea . The protein shells of non-enveloped viruses including poliovirus [33] , human papillomavirus [34] , [35] , common cold viruses [6] , [31] and many others are built from many copies of some few different proteins. Similarly, Rickettsia prowazekii , R. typhii , the cause of typhus [36] , and B. anthracis , the causative agent of anthrax [37] and numerous other human and animal bacterial pathogens [10] , [38] carry highly repetitive structures in the form of S-layers. Such S-layers have been frequently used for the presentation of foreign epitopes in vaccines, in immunotherapy of cancers, and in antiallergic immunotherapy [10] . Recently, this approach was followed to elicit a broader and more potent immunity against H1N1 as compared with the traditional influenza vaccines [39] . In this study, the viral hemagglutinin was genetically fused to ferritin, a protein that naturally forms small protein crystals composed of 24 identical polypeptides. Here, we demonstrate bipedal walking of antibodies on surface lattices very similar to such vaccines and immunogens. We propose that antibody locomotion underlies the following mechanism ( Fig. 3 ); steric strain (stored in elasticity and/or, linear and rotational distortions of either the IgG and/or the substrate which cannot be fully compensated for by the antibodies hinge region) reduces the strength of the bonds between a bivalently bound IgG molecule and its two cognate epitopes effectively reducing the antibody/antigen dissociation energy barrier. Therefore, for antibodies stochastically moving on rigid 2D protein crystals, each of the two single bonds can dissociate faster when compared with the unique single bond of a Fab molecule; the free Fab leg then rebinds to the same or to another antigen nearby generating a single step-like move. Moving speeds and step sizes are thus dictated by steric constraints driving the dissociation and reassociation of just one leg at a time; the mechanism results in clustering as required for complement binding and phagocytosis [9] . It is likely that similar effects also drive aggregation of mobile multivalent membrane proteins by bivalent interaction partners; when a suboptimal distance and/or geometric constraint does not allow for stable bidentate binding, the dynamic dissociation of one of the paratopes will favour attachment to an epitope on a second mobile antigen nearby ultimately resulting in crowding. Such a mechanism might be involved in the fine-tuning of signal transduction and cell adhesion. Besides these biological aspects, our findings will inspire the rational design of antibodies and multivalent receptors based on polypeptides and bio-mimetic nanomaterials to exploit/inhibit steric strain-induced dynamic effects for tunable surface recognition and adhesion [1] . HS-AFM apparatus and cantilevers High-speed AFM [13] was operated in tapping mode at room temperature (25 °C) with free amplitudes of 1.5–2.5 nm and an amplitude set point of larger than 90%. Silicon nitride cantilevers, (BL-AC10DS-A2, Olympus, Tokyo, Japan) with nominal spring constants of 0.1 N m −1 , a resonance frequency of ~500 kHz, and a quality factor of ~2 in liquids were used. Sample preparation Mutant Sendai PM and HRV2 were produced and prepared for imaging on Mica as described [5] , [40] . S-layer fusion proteins rSbpA-Strep-tag II were produced and recrystallized on clean silicon wafers as described [23] . Streptavidin 2D crystals were formed on a supported lipid bilayer (DOPC, DOPS, biotin-cap-DOPE; weight ratio of 7:2:1) deposited on mica as described [26] . Anti-Sendai (MAb VII-E-7) [20] , anti-Strep-tag II (StrepMAb-Immo) [24] (IBA, Goettingen, Germany), and anti-Streptavidin (Fisher Scientific, Vienna, Austria) antibodies were used at a final concentration of ~50 μg ml −1 , mAbs 8F5 and 3B10 against HRV2 were used at a final concentration of ~10 μg ml −1 , respectively. StrepMAb-Immo-Fabs were produced using a Fab preparation kit (Pierce Biotechnology, Rockford, IL, USA) and used at a final concentration of ~9 μg ml −1 . Image and trajectory analysis Images were analysed using ImageJ (NIH) with a plug-in for multiple particle detection and tracking (ParticleTracker v. 1.5 (ref. 41) [41] ). Trajectories were further processed using in-house algorithms implemented in MATLAB (MathWorks). The distribution of step sizes was determined using threshold analysis, accounting for the fluctuations in positional accuracy due to the diffuse location of the free rotating Fc fragments of the antibodies. Only steps (and corresponding dwell times) larger than a threshold of 2 nm (as determined in a separate experiment, Fig. 2e ) were analysed and collected for the histograms in Fig. 2 . The dwell time distributions were cumulatively summed, normalized and fitted by a single exponential distribution, 1−exp(− t / τ ), yielding the characteristic time constant τ for each experiment. The mean square displacement was calculated as a function of the time−lag t lag . Lateral diffusion constants D were determined according to (ref. 42 ), with σ xy specifying the localization precision. Epitope spacings and orientations Since crystal structures of the epitope–paratope complexes used in our studies were not available, the exact orientation of epitopes and paratopes are not known. We thus assessed the number and symmetry relations of epitope pairs that are accessible for bivalent antibody binding as follows: from the well-known crystal parameters and positions of epitopes [21] , [22] , the intrinsic symmetry relations between epitope pairs depicted in Fig. 3e,k where computed by first arbitrarily assigning an intrinsic orientation (marked as arrow) to a centre epitope. The orientation of the neighbouring epitopes was calculated using the respective crystal symmetries and lattice constants. Then, a diagram showing the relative orientations of individual epitopes pairs with respect to each other was generated. Comparison with the X-ray structure of HRV2 Surface features at the three icosahedral symmetry axes of a virion are displayed in Fig. 5 ; PDB:1FPN X-ray coordinates were converted into a volume by using electron scattering form factors followed by Fourier-filtering to 20 Å with xmipp [43] . Images were rendered with Chimera [44] at a threshold of 1 σ . In all views only the uppermost 19 Å of the volume are displayed. How to cite this article: Preiner, J. et al. IgGs are made for walking on bacterial and viral surfaces. Nat. Commun. 5:4394 doi: 10.1038/ncomms5394 (2014).